Tailoring deposition and morphology of discharge products towards high-rate and long-life lithium-oxygen batteries Lithium-oxygen batteries are an attractive technology for electrical energy storage because of their exceptionally high-energy density; however, battery applications still suffer from low rate capability, poor cycle stability and a shortage of stable electrolytes. Here we report design and synthesis of a free-standing honeycomb-like palladium-modified hollow spherical carbon deposited onto carbon paper, as a cathode for a lithium-oxygen battery. The battery is capable of operation with high-rate (5,900 mAh g −1 at a current density of 1.5 A g −1 ) and long-term (100 cycles at a current density of 300 mA g −1 and a specific capacity limit of 1,000 mAh g −1 ). These properties are explained by the tailored deposition and morphology of the discharge products as well as the alleviated electrolyte decomposition compared with the conventional carbon cathodes. The encouraging performance also offers hope to design more advanced cathode architectures for lithium-oxygen batteries. The pressing concerns of reducing greenhouse gas emissions and the consumption of non-renewable fossil fuels have led to increased demands for electrochemical energy storage systems with energy densities that far exceed those of lithium-ion batteries [1] . To this end, rechargeable lithium-oxygen (Li-O 2 ) batteries have been the focus of great interest because of their extremely high energy potentiality (up to 2–3 kWh kg −1 ) because oxygen, the cathode material, is not necessarily stored in batteries, as with the convention lithium-ion battery technology, but can be accessed from the environment [2] , [3] , [4] , [5] . A typical rechargeable non-aqueous Li-O 2 cell is composed of a Li metal anode, a non-aqueous Li + conducting electrolyte, and a porous cathode. Theoretically, the electrochemical reaction is 2Li + +2e − +O 2 ⇆ Li 2 O 2 , with the forward direction describing the discharge of the cell and the reverse direction describing the charge [6] . However, in practice, the system has presented many scientific and technological challenges since it was introduced in 1996 (ref. 7 ). The decomposition of the organic electrolytes during the discharge and charge processes causes the battery instability and electrolyte depletion [8] , [9] , [10] , [11] . The irregular precipitation of thick film-like or large toroid-like insoluble discharge product, lithium peroxide (Li 2 O 2 ), blocks the void of the O 2 cathode and eventually limits the battery performance, including the specific capacity, charge efficiency and cycle life [12] , [13] , [14] , [15] . The continuous accumulation of lithium carbonate (Li 2 CO 3 ) and lithium carboxylates, resulting from side reactions of the Li 2 O 2 and intermediate species, such as LiO 2 * and O 2 − , with the cathode and the electrolyte on cycling, leads to cathode passivation and battery death [16] , [17] , [18] . The insufficient structural stability of the cathode during Li 2 O 2 formation/decomposition is also a limitation for battery cycle life [19] , [20] . In response, previous studies have reported that these limitations can be partially overcome by employing a sophisticated cathode, reducing the discharge/charge overpotentials to alleviate electrolyte decomposition [21] , tailoring the deposition site and morphology of Li 2 O 2 within cathode to enhance the specific capacity, charge efficiency, and cycle life [22] , [23] , [24] and tuning the porous structure of the cathode to improve cycle stability [20] . Although much progress has been achieved, the improvements are still far from overcoming the many limitations, such as poor rate capability, low cycle stability and poor energy efficiency, which still prevent the practical implementation of the Li-O 2 battery [25] , [26] . Therefore, there is an urgent need to design and fabricate a highly efficient cathode. In principle, an ideal cathode for a non-aqueous Li-O 2 battery should possess many critical properties, including high electrical conductivity for electron transfer, optimized porous structure to ensure accommodation of a large amount of discharge products and to facilitate rapid mass (oxygen and lithium ions) transportation, high catalytic activity and selectivity for catalysing the 2Li + +2e − +O 2 ⇆ Li 2 O 2 reaction, and good structural integrity. Here we develop a strategy by combining electrophoresis with template replication to fabricate a free-standing palladium (Pd)-modified hollow spherical carbon deposited onto carbon paper cathode (P-HSC deposited onto CP) with a tailored hierarchically porous honeycomb-like structure, which endows the Li-O 2 battery with a high specific capacity, relatively low overpotentials and superior rate capability. Further, we show that the Pd nanocrystals (NPs) on the wall within the free-standing hollow carbon spheres facilitate the formation of isolated nanosheets of Li 2 O 2 , thus resulting in a rapid and stable electrochemical Li-O 2 reaction. We suggest that the obtained superior performance is primarily the result of the hierarchically porous structure, the high catalytic activity and the surface nature of the P-HSC deposited onto CP cathode. This strategy might contribute to improve lithium–air battery technology. 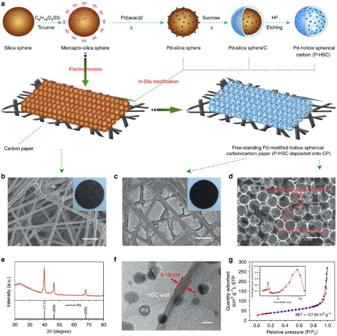Figure 1: Scheme for fabrication and structure of the cathode. (a) Schematic representations for the design and preparation of the palladium (Pd)-modified hollow spherical carbon (P-HSC) deposited onto carbon paper (CP) cathode. (b) The field emission scanning electron microscopic (FESEM) image and photograph (inset) of the pristine CP. Scale bars, 50 μm. (c) FESEM image and photograph (inset) of the as-prepared P-HSC deposited onto CP cathode. Scale bars, 50 μm. (d) The enlarged image ofc. Scale bars, 500 nm. The red arrows indpoint out the hierarchically porous structure of P-HSC deposited onto CP. (e) X-ray diffraction patterns of the as-prepared P-HSC and the standard pattern of Pd nanocrystals. (f) TEM image of the P-HSC. The inner wall surface of the hollow carbon spheres (light area) is covered with well-dispersed Pd NPs with 10–15 nm in diameter (dark areas). Scale bars, 10 nm. (g) Nitrogen adsorption-desorption isotherms and pore-size distribution (inset) of the P-HSC. Synthesis and analysis of P-HSC deposited onto CP O 2 cathode Figure 1a shows the synthesis strategy for the P-HSC deposited onto CP cathode. First, mercaptopropylsilyl-functionalized silica spheres (MPS-SS) are deposited into the framework of the CP (MPS-SS deposited onto CP) using an electrophoretic technique. Then, the sample is in situ -loaded with Pd NPs and covered with a carbon shell. The morphology and porous structure of the P-HSC deposited onto CP cathode are investigated by field emission scanning electron microscopy and transmission electron microscopy (TEM). As shown in Fig. 1b,c , without the help of any additional binder or solvent, the P-HSC is firmly embedded into the framework of the CP, which ensures the formation of a free-standing structure and a favourable low-resistance pathway for electron transfer. High-magnification observation ( Fig. 1d ) of the P-HSC deposited onto CP cathode reveals that the P-HSC consist of numerous open hollow spherical macropores of ~500 nm in diameter and ~9 nm in wall thicknesses ( Fig. 1f ). These P-HSC are interconnected through open windows with ~20–100 nm in diameter throughout the entire cathode, leading to a honeycomb-like pore structure. The powder X-ray diffraction (PXRD) analysis of the P-HSC ( Fig. 1e ) reveals that the diffraction peaks can be indexed to well-crystallized Pd NPs (PDF No. 46–1,043). The TEM images ( Fig. 1f and Supplementary Fig. S1a ) reveal that the Pd NPs with 10–15 nm diameters (dark areas) are well-dispersed on the wall surface of the hollow carbon spheres (light area) and their content is ~25 wt% ( Supplementary Fig. S2 ). The N 2 -adsorption isotherm and the pore-size distribution are shown in Fig. 1g . The N 2 -adsorption isotherm of the P-HSC exhibits the combined characteristics of type I/II [27] , [28] , with a surface area of 127 m 2 g −1 and a total pore volume of 0.22 cm 3 g −1 . The initial region of the isotherms experiences a slight rise at low P/P 0 , indicating the presence of micropores, and a hysteresis loop in the P/P 0 range of 0.4–1.0 is indicative of mesoporosity. From the pore-size distribution, it is clearly observed that there are two kinds of pores: micropores (~3 nm) and mesopores with a wide size range (20–100 nm), which is in agreement with the scanning electron microscopy (SEM) results ( Fig. 1d ). The obtained P-HSC deposited onto CP has many tailored properties, which are vital to the transportation of electrons, ions and oxygen, and consequently, the oxygen reduction (ORR) and evolution reactions (OER) of the Li-O 2 battery. The high-conductive CP and the embedded spherical carbon facilitate the continuous and high flux of electron transfer throughout the cathode. The interconnected pores offer sufficient channels to transfer O 2 , electrolyte and reaction intermediate species freely to/from the inner cathode, ensuring uniform reactant distributions and adequate triphase regions required for the ORR and OER. The large hollow volume within the P-HSC deposited onto CP provides enough place for the deposition/decomposition of the discharge products. The Pd NPs can control the deposition behaviour and morphology of the discharge product to enhance the Li-O 2 reaction. The structural stability of the CP and the embedded free-standing structure help to maintain stable cathode integrity upon cycling. All of these advantages benefit the electrochemical performance of the Li-O 2 battery. Figure 1: Scheme for fabrication and structure of the cathode. ( a ) Schematic representations for the design and preparation of the palladium (Pd)-modified hollow spherical carbon (P-HSC) deposited onto carbon paper (CP) cathode. ( b ) The field emission scanning electron microscopic (FESEM) image and photograph (inset) of the pristine CP. Scale bars, 50 μm. ( c ) FESEM image and photograph (inset) of the as-prepared P-HSC deposited onto CP cathode. Scale bars, 50 μm. ( d ) The enlarged image of c . Scale bars, 500 nm. The red arrows in d point out the hierarchically porous structure of P-HSC deposited onto CP. ( e ) X-ray diffraction patterns of the as-prepared P-HSC and the standard pattern of Pd nanocrystals. ( f ) TEM image of the P-HSC. The inner wall surface of the hollow carbon spheres (light area) is covered with well-dispersed Pd NPs with 10–15 nm in diameter (dark areas). Scale bars, 10 nm. ( g ) Nitrogen adsorption-desorption isotherms and pore-size distribution (inset) of the P-HSC. Full size image Properties of the P-HSC deposited onto CP cathode The electrochemical properties of the P-HSC deposited onto CP cathode were then examined in a Li-O 2 cell. The free-standing HSC deposited onto CP cathode and conventional Super P carbon (SP) cathode were employed for comparison ( Supplementary Fig. S3 ). Lithium triflate (LiCF 3 SO 3 ) in tetraethylene glycol dimethyl ether (TEGDME) was employed as the electrolyte because of its relatively higher stability towards superoxide (O 2 − ) (refs 3 , 29 , 30 ). All of the results for the specific capacities and current densities are calculated with the total carbon mass in the O 2 cathodes. 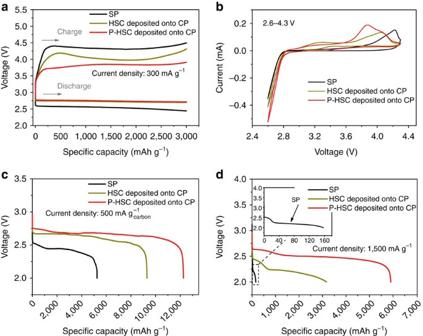Figure 2: Electrochemical performance. (a) First charge–discharge curves of lithium-oxygen (Li-O2) cells at a current density of 300 mA g−1and a specific capacity limit of 3,000 mAh g−1. (b) CV of the three kinds of cathode in Li-O2cells at a constant scan rate of 0.1 mV s−1. (c) The rate capability of the Li-O2cells with the three kinds of cathode at the current density of 500 mA g−1. (d) The rate capability of the Li-O2cells with the three kinds of cathode at the current density of 1,500 mA g−1. Inset indis the enlarged discharge profile of the Li-O2cells with conventional Super P carbon (SP) cathode. Figure 2a shows the first discharge (ORR)-charge (OER) voltage profiles of the Li-O 2 cells with P-HSC deposited onto CP, HSC deposited onto CP and SP cathodes at a current density of 300 mA g −1 . The discharge and charge voltage of the Li-O 2 cell can be significantly improved with the help of the P-HSC deposited onto CP cathode, which enhances the round-trip efficiency (the ratio of discharge to charge voltage) that is vital for electrochemical energy storage devices. In detail, the discharge voltage of the Li-O 2 cell with a P-HSC deposited onto CP cathode is higher than that with the HSC deposited onto CP by ~30 mV and SP by ~190 mV. Its charge voltage is much lower than that with the HSC deposited onto CP cathode by 170 mV and SP by 300 mV. This result is further supported by the oxidation of the artificially Li 2 O 2 -loaded electrodes in Li-O 2 cells, which indicates that a similar reduction in the oxidation potential is obtained ( Supplementary Fig. S4 ). The electrochemical processes of oxygen in the Li-O 2 cell were also investigated using cyclic voltammetry (CV). Figure 2b presents the CV response of the cells at a constant scan rate of 0.1 mV s −1 . The first cycle curve reveals that the P-HSC deposited onto CP cathode exhibits a higher current density compared with the HSC deposited onto CP and SP cathodes. These results show that the P-HSC deposited onto CP exhibits superior electrochemical performance towards both formation and decomposition of discharge product, which might be derived from the synergy of the following advantageous factors: the large Brunaure–Emmert–Teller surface area and substantial surface defects ( Supplementary Fig. S5 ) that provide more reaction sites for the ORR and OER; the hierarchically porous structure and Pd NPs modification, which facilitate the continuous oxygen and lithium ion flow into/departure from the inner cathode via larger tunnels and the triphase reaction catalysed by both nanoscale carbon pores and Pd nanocrystals [31] , [32] ; and the well-tailored deposition behaviour and morphology of the discharge product that benefits the ORR and OER reactions ( vide infra ). Figure 2: Electrochemical performance. ( a ) First charge–discharge curves of lithium-oxygen (Li-O 2 ) cells at a current density of 300 mA g −1 and a specific capacity limit of 3,000 mAh g −1 . ( b ) CV of the three kinds of cathode in Li-O 2 cells at a constant scan rate of 0.1 mV s −1 . ( c ) The rate capability of the Li-O 2 cells with the three kinds of cathode at the current density of 500 mA g −1 . ( d ) The rate capability of the Li-O 2 cells with the three kinds of cathode at the current density of 1,500 mA g −1 . Inset in d is the enlarged discharge profile of the Li-O 2 cells with conventional Super P carbon (SP) cathode. Full size image Further evidence for the P-HSC deposited onto CP leading to improvement of the Li-O 2 cell comes from the very low interfacial resistance of 50.3 Ω cm −2 between the electrolyte and the P-HSC deposited onto CP cathode ( Supplementary Fig. S6 ), which encouraged us to further investigate the rate performance of the Li-O 2 cell. Figure 2c,d and Supplementary Fig. S7 show the first discharge curves of the Li-O 2 cells with the P-HSC deposited onto CP, HSC deposited onto CP and SP cathodes at current densities of 500, 1,000 and 1,500 mA g −1 , respectively. It can be seen that, at the current density of 500 mA g −1 , the Li-O 2 cell with the P-HSC deposited onto CP cathode exhibits a higher discharge capacity of 12,254 mAh g −1 than those with the HSC deposited onto CP (9,280 mAh g −1 ) and the SP (5,250 mAh g −1 ). Unexpectedly, even at the very high current density of 1,500 mA g −1 , the discharge capacity of the P-HSC deposited onto CP can still reach 5,900 mAh g −1 , which is more than 37 times than that with the conventional SP cathode (160 mAh g −1 ), which is among the best rate performances of non-aqueous Li-O 2 batteries [3] , [16] , [24] , [27] , [33] . It should be noted that the discharge/charge capacity of the Li-O 2 cells using only a pristine CP cathode is very low ( Supplementary Fig. S8 ), indicating that P-HSC brings about the high discharge/charge capacity. Similarly, it is found that the background discharge capacity of the Ar-filled cells is negligible within the voltage range, which suggests that the discharge capacities of Li-O 2 cells are derived from ORR ( Supplementary Fig. S9 ). These improvements to the specific capacity and rate capability of Li-O 2 cells further confirm the advantages of the P-HSC deposited onto CP, which might be attributed to the synergistic effect of the high ORR and OER activities and the tailored hierarchically porous structure of the P-HSC deposited onto CP. The plentiful large pores of the P-HSC deposited onto CP provide enough void volume for the discharge product deposition, and thus result in a much enhanced discharge capacity, whereas the difference in the specific capacities of the P-HSC deposited onto CP and HSC deposited onto CP comes from the different deposition behaviour and morphology of the discharge product ( vide infra ). In general, charge transfer is the rate-determining process at low current densities. However, when the current density increases, the mass transfer of lithium ions and oxygen could become the rate-determining process. Uniform oxygen and lithium ion distribution inside the P-HSC deposited onto CP cathode is required to improve the rate capability, especially at very high current density [34] . Minimal interfacial resistance is also beneficial to the high rate capability. Another considerable improvement of the Li-O 2 cell with P-HSC deposited onto CP is the cycling stability. Following the recently widely used capacity-limited cycle method [3] , Fig. 3 presents the typical voltage profiles for Li-O 2 cells with P-HSC deposited onto CP, HSC deposited onto CP and SP cathodes cycled at a rate of 300 mA g −1 and a fixed capacity of 1,000 mAh g −1 . The voltage obtained at the discharge terminal of the P-HSC deposited onto CP cathode in the Li-O 2 cell is >2.0 V for 205 cycles ( Fig. 3a,b ). In contrast, the discharge voltages of the HSC deposited onto CP and SP cathodes degraded to <2.0 V after only 125 and 43 cycles, respectively ( Fig. 3c–f ). We extended the battery test by determining the cycling response under different specific capacity limits. As shown in Supplementary Fig. S10a,b , 61 and 33 stable cycles were obtained with capacities of 2,000 and 5,000 mAh g −1 , respectively, further corroborating the good stability of the Li-O 2 cell with the P-HSC deposited onto CP cathode, even at high capacity, which is among the best cycling performances reported to date in this field [3] , [35] , [36] . In addition to the high catalytic activity of the P-HSC deposited onto CP cathode, its unique hierarchical porous structure and the nanosheet-shaped structure of Li 2 O 2 ( Fig. 4c ), which ensures a uniform oxygen and electrolyte distribution around the discharge products, promote the decomposition of the products during charge and result in an enhancement of the rechargeability. Further, the high durability of the free-standing structure of the P-HSC deposited onto CP ( Fig. 5b ) also contributes to the high cycling stability. 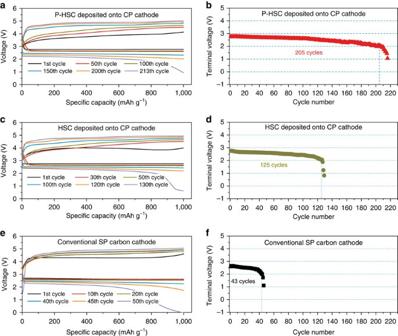Figure 3: Battery cycling stability. (a) Discharge–charge curves of the Li-O2cells with the P-HSC deposited onto CP cathode at different cycles. (b) Variation of voltage on the terminal of discharge of the Li-O2cells with the P-HSC deposited onto CP cathode. (c) Discharge–charge curves of the Li-O2cells with the HSC deposited onto CP cathode at different cycles. (d) Variation of voltage on the terminal of discharge of the Li-O2cells with the HSC deposited onto CP cathode. (e) Discharge–charge curves of the Li-O2cells with the conventional SP cathode at different cycles. (f) Variation of voltage on the terminal of discharge of the Li-O2cells with the SP cathode. Figure 3: Battery cycling stability. ( a ) Discharge–charge curves of the Li-O 2 cells with the P-HSC deposited onto CP cathode at different cycles. ( b ) Variation of voltage on the terminal of discharge of the Li-O 2 cells with the P-HSC deposited onto CP cathode. ( c ) Discharge–charge curves of the Li-O 2 cells with the HSC deposited onto CP cathode at different cycles. ( d ) Variation of voltage on the terminal of discharge of the Li-O 2 cells with the HSC deposited onto CP cathode. ( e ) Discharge–charge curves of the Li-O 2 cells with the conventional SP cathode at different cycles. ( f ) Variation of voltage on the terminal of discharge of the Li-O 2 cells with the SP cathode. 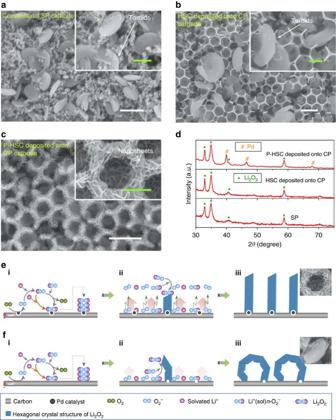Figure 4: Morphology and deposition mechanism. (a) Field emission scanning electron microscopic (FESEM) images of the discharged SP cathode when the discharge capacity is limited to 3,000 mAh g−1. White scale bars, 1 μm. Green scale bars, 400 nm. (b) The FESEM images of the discharged HSC deposited onto CP cathode. White scale bars, 1 μm. Green scale bars, 400 nm. (c) The images of the discharged P-HSC deposited onto CP cathode. White scale bars, 1 μm. Green scale bars, 400 nm. The insets ina–care the corresponding enlarged FESEM images. (d) Corresponding PXRD patterns of the three kinds of discharged cathode. It is found that the PXRD peaks can be assigned to Li2O2, although the morphology of the discharge product is different. (e) A mechanism for the electrochemical production of Li2O2nanosheet-like aggregates on P-HSC deposited onto CP cathode. (f) A mechanism for the electrochemical production of Li2O2toroidal aggregates on SP and HSC deposited onto CP cathodes. The panelsiineandfillustrate the nucleation processes of Li2O2. The panelsiiineandfillustrate that the small elongated hexagonal nanocrystallites come into being after the nucleation of Li2O2. The Li2O2preferentially nucleates and grows on the prismatic crystal faces. The panelsiiiineandfillustrate the formation of the observed toroidal and nanosheet-like aggregates. Full size image Figure 4: Morphology and deposition mechanism. ( a ) Field emission scanning electron microscopic (FESEM) images of the discharged SP cathode when the discharge capacity is limited to 3,000 mAh g −1 . White scale bars, 1 μm. Green scale bars, 400 nm. ( b ) The FESEM images of the discharged HSC deposited onto CP cathode. White scale bars, 1 μm. Green scale bars, 400 nm. ( c ) The images of the discharged P-HSC deposited onto CP cathode. White scale bars, 1 μm. Green scale bars, 400 nm. The insets in a – c are the corresponding enlarged FESEM images. ( d ) Corresponding PXRD patterns of the three kinds of discharged cathode. It is found that the PXRD peaks can be assigned to Li 2 O 2 , although the morphology of the discharge product is different. ( e ) A mechanism for the electrochemical production of Li 2 O 2 nanosheet-like aggregates on P-HSC deposited onto CP cathode. ( f ) A mechanism for the electrochemical production of Li 2 O 2 toroidal aggregates on SP and HSC deposited onto CP cathodes. The panels i in e and f illustrate the nucleation processes of Li 2 O 2 . The panels ii in e and f illustrate that the small elongated hexagonal nanocrystallites come into being after the nucleation of Li 2 O 2 . The Li 2 O 2 preferentially nucleates and grows on the prismatic crystal faces. The panels iii in e and f illustrate the formation of the observed toroidal and nanosheet-like aggregates. 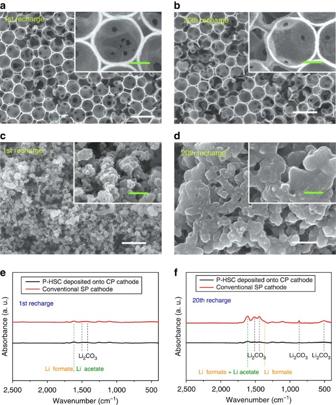Figure 5: Cathode rechargeability. (a,b) Field emission scanning electron microscopic (FESEM) images of the recharged P-HSC deposited onto CP cathode after the 1st and 20th cycle. White scale bars, 1 μm. Green scale bars, 200 nm. (c,d) FESEM images of the recharged SP cathode after the 1st and 20th cycle. White scale bars, 1 μm. Green scale bars, 400 nm. Insets ofa–dshow the corresponding enlarged FESEM images. The current density is 300 mA g−1and the specific capacity is 3,000 mAh g−1. (e,f) Corresponding FTIR spectra of two kinds of recharged cathode after the 1st and 20th cycle. Full size image Figure 5: Cathode rechargeability. ( a , b ) Field emission scanning electron microscopic (FESEM) images of the recharged P-HSC deposited onto CP cathode after the 1st and 20th cycle. White scale bars, 1 μm. Green scale bars, 200 nm. ( c , d ) FESEM images of the recharged SP cathode after the 1st and 20th cycle. White scale bars, 1 μm. Green scale bars, 400 nm. Insets of a – d show the corresponding enlarged FESEM images. The current density is 300 mA g −1 and the specific capacity is 3,000 mAh g −1 . ( e , f ) Corresponding FTIR spectra of two kinds of recharged cathode after the 1st and 20th cycle. Full size image Morphology and deposition mechanism of the Li 2 O 2 To further understand the obtained superior behaviour of the P-HSC deposited onto CP cathode in a Li-O 2 cell, the morphologies of the cathodes at different discharge-recharge stages were examined. Figure 4a–c show the SEM images of the discharged SP, HSC deposited onto CP and P-HSC deposited onto CP cathodes at a fixed capacity of 3,000 mAh g −1 . The morphologies of the discharge products are completely different even under same discharge current density of 300 mA g −1 . The discharge product on the SP and HSC deposited onto CP cathodes is toroidal and irregularly dispersed, which is consistent with the results obtained by other groups [13] , [15] . In sharp contrast, unique nanosheets with <10 nm thicknesses uniformly grew onto the wall of the hollow carbon spheres of the P-HSC deposited onto CP cathode. PXRD analysis of the discharged cathodes confirmed that Li 2 O 2 is the only crystalline product in the three cases, regardless of the difference in the morphology of the discharge product ( Fig. 4d ). The high packing density of the toroid-shaped Li 2 O 2 hinders the formation of the Li 2 O 2 –electrolyte interface that supports the electrochemical reaction during the charge process and consequently degrades the charge performance of the Li-O 2 battery with the SP and HSC deposited onto CP cathodes. In contrast, for the P-HSC deposited onto CP cathode, the uniformly and loosely distributed Li 2 O 2 nanosheets provide sufficient Li 2 O 2 –electrolyte interfaces, leading to enhanced rechargeability of the Li-O 2 cell, which is further supported by the SEM results of the recharged cathode ( Fig. 5a,b ). Figure 4e,f schematically show the mechanism of electrochemical growth of the Li 2 O 2 nanosheets and toroids. The first step is the binding of O 2 to the cathode surface, especially with carbon defect sites and Pd catalysts, followed by the reduction to form O 2 − , which binds with Li + to form LiO 2 * (refs 37 , 38 ). The LiO 2 * can either desorb by solvation [39] and undergo a disproportionation reaction (2LiO 2 *→Li 2 O 2 +O 2 ) [40] near the surface of the cathode to form Li 2 O 2 or undergo direct reduction with Li + /e − to form Li 2 O 2 (LiO 2 *+e − +Li + →Li 2 O 2 ; panel i in Fig. 4e,f ) [41] . At a critical concentration, small elongated hexagonal nanocrystallites appear after the nucleation of the Li 2 O 2 (panel ii in Fig. 4e,f ) [42] . The strong binding of superoxide (O 2 − or LiO 2 *) with the carbon defect sites traps the superoxide on the cathode surface (a short diffusion path), leading to a poor superoxide availability on the prismatic crystal faces (a preferred nucleation site) and gives rise to the observed toroid aggregates for Li 2 O 2 (panel iii in Fig. 4f ). In contrast, in the P-HSC deposited onto CP cathode, the Pd nanocrystal surfaces are considered to be less ‘sticky’ than carbon surfaces riddled with dangling bonds [43] , which can weaken the binding of the generated superoxide to the substrate, thus enhancing the diffusion of the superoxide molecules away from the cathode surface (panel iii in Fig. 4e ), favoring the nucleation and crystallization of Li 2 O 2 on the preferred prismatic crystal faces and leading to nanosheet-shaped structure growth (panel iii in Fig. 4e ). However, the low overpotential measured above ( Fig. 2a ) indicates that more active sites on the P-HSC deposited onto CP cathode are formed under the catalysis of the Pd NPs, which might also contribute to the homogeneous distribution of the O 2 − or LiO 2 * close to the cathode surface, beneficial to nanosheet formation. However, in a real system, Li 2 O 2 growth is more complicated and further studies using a combination of electrochemical and theoretical approaches are in progress to elucidate the exact functions of Pd in the growth of the Li 2 O 2 nanosheets. Reversibility of P-HSC deposited onto CP cathode To further examine the stability of the P-HSC deposited onto CP cathode in a Li-O 2 cell upon cycling, the morphology changes of the recharged O 2 cathodes after the 1st and 20th cycle were examined. The nanosheet-shaped discharge products disappeared, and the hierarchically porous honeycomb-like structure of the whole cathode almost fully recovered, even after the 20th charge, indicating good structure reversibility and stability of the P-HSC deposited onto CP cathode, which contributes to the high cycling stability ( Fig. 3a,b ). Even after 20 cycles, the inner wall of the hollow carbon spheres for the recharged P-HSC deposited onto CP cathode is only covered by thin films or small particles (inset of Fig. 5b ), which can be assigned as Li 2 CO 3 , HCO 2 Li or lithium acetate (CH 3 CO 2 Li) from the side reactions of the Li 2 O 2 and/or intermediates such as LiO 2 *, carbon surface and especially electrolyte [44] , [45] on cycling ( Fig. 5e ). In contrast, in the conventional SP carbon cathode, massive Li 2 CO 3 and lithium carboxylates packed densely onto the cathode surface ( Fig. 5d,f ). This continuous accumulation of Li 2 CO 3 and lithium carboxylates upon cycling hinders the transportation of the superoxide species, electrons and lithium ions within the cathode during subsequent cycling, which consequently leads to the failure of the Li-O 2 cell with a conventional carbon cathode. These results further confirm the superiority of the P-HSC deposited onto CP cathode in terms of rechargeability and stability. First, the unique nanosheet-shaped Li 2 O 2 on the P-HSC deposited onto CP is easily decomposed on recharge. Second, the P-HSC deposited onto CP cathode significantly alleviates the high-potential-induced electrolyte decomposition during charge by the lowered charge voltage and/or decreased reactivity of the released nascent O 2 (refs 43 , 45 ). The superior rechargeability of the P-HSC deposited onto CP cathode was further examined by the PXRD technique ( Fig. 6 ). In the conventional SP carbon cathode, although the discharge products at the end of the 1st discharge are dominated by crystalline Li 2 O 2, crystalline Li 2 O 2 becomes barely visible and cannot be detected after 10 and 20 cycles ( Fig. 6a ), respectively, which is similar to previously reported results [29] . In contrast, in the P-HSC deposited onto CP cathode, there is clear evidence of crystalline Li 2 O 2 even after 20 cycles ( Fig. 6b ). We speculate that the degradation of the crystalline Li 2 O 2 on cycling could be ascribed to both the increasing accumulation of the abovementioned Li 2 CO 3 and lithium carboxylates on the cathode surface and the presence of CO 2 in the electrolyte (from the electrochemical oxidation of the Li 2 CO 3 and lithium carboxylates during charging), which inhibit the nucleation and crystallization of Li 2 O 2 during the subsequent discharge, leading to the formation of amorphous Li 2 O 2 . Although the exact underlying mechanism is not yet clear, the differences in the stability of Li 2 O 2 on cycling indicate that the P-HSC deposited onto CP cathode could suppress the formation of the Li 2 CO 3 and lithium carboxylates on cycling, which is in agreement with the SEM results ( Fig. 5 ), resulting in a favourable rechargeability and a good stability of the Li-O 2 cell. 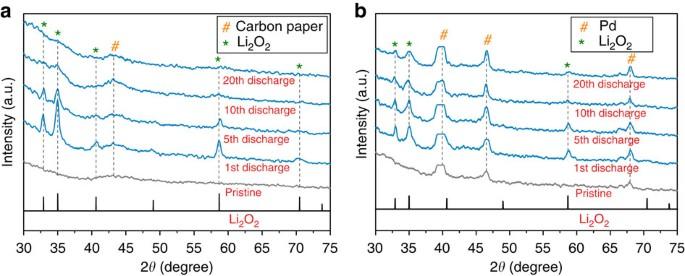Figure 6: Product reversibility. (a) PXRD patterns of discharge products on conventional SP at the end of discharge after the indicated number of cycles. (b) P-HSC deposited onto CP cathode. The current density is 300 mA g−1and the discharge–charge specific capacity is 1,000 mAh g−1. Figure 6: Product reversibility. ( a ) PXRD patterns of discharge products on conventional SP at the end of discharge after the indicated number of cycles. ( b ) P-HSC deposited onto CP cathode. The current density is 300 mA g −1 and the discharge–charge specific capacity is 1,000 mAh g −1 . Full size image These experimental results show that the cathode can tailor the deposition behaviour and morphology of Li 2 O 2 and alleviate long-term decomposition of TEGDME, consequently improving the electrochemical performance of the Li-O 2 battery. However, investigation into the process of Li 2 O 2 formation and decomposition is crucial for the understanding of the electrochemical behaviour in the Li-O 2 battery. The XRD patterns in Fig. 6 show qualitative evidence that Li 2 O 2 is formed with the P-HSC deposited onto CP and conventional SP carbon cathodes. However, the PXRD is only qualitative and blind to the likely amorphous electrolyte decomposition products (carboxylates, and so on). In response, in addition to the electrochemical and morphological characterization, we attempted to look quantitatively at the Li-O 2 chemistry, for example, how much Li 2 O 2 is formed on discharge. To this end, following the recently developed method [36] , Fourier transform infrared (FTIR) calibration curves were obtained by mixing known amounts of Li 2 O 2 with Li 2 CO 3 , Li 2 O 2 with CH 3 CO 2 Li and Li 2 O 2 with lithium formate (HCO 2 Li) with varying ratios ( Supplementary Figs S11–S13 ). On the basis of these calibration curves, the molar ratio of Li 2 O 2 , Li 2 CO 3 , CH 3 CO 2 Li and HCO 2 Li in the discharge products was determined from the obtained FTIR spectra ( Fig. 7 ), which are tabulated in Supplementary Tables S1 and S2 and Supplementary Fig. S14 . The quantitative FTIR results show that the proportion of Li 2 O 2 in product after 1, 20, 40, 100 and 200 cycles is 95.6%, 91.0%, 81.6%, 70.5% and 43.6%, respectively. The large amount of Li 2 O 2 formed on discharge could reasonably exclude the possibility that the cycling was simply because of the irreversible decomposition of the electrolyte in the battery. In sharp contrast, the proportion of Li 2 O 2 at the end of 40 cycles for the Li-O 2 battery with the SP cathode was only 41.3%, which is much lower than that with the P-HSC deposited onto CP cathode (81.6%). This might also exclude the possibility that the infrared observation of fewer electrolyte decomposition products in the cathode after charging ( Fig. 5e,f ) is simply because Pd catalyses the charging of the electrolyte decomposition products. In addition, 1 H nuclear magnetic resonance (NMR) spectroscopy ( Supplementary Figs S15 and S16 ) demonstrated that the amount of electrolyte decomposition product on the P-HSC deposited onto CP cathode was less than that on the SP cathode on cycling, which is consistent with the above quantitative FTIR results. As a supplement to XRD, both quantitative FTIR and NMR results are in good agreement with the electrochemical behaviour of the Li-O 2 battery, which confirms the superiority of the P-HSC deposited onto CP cathode in terms of alleviating the long-term decomposition of TEGDME by tailoring the deposition behaviour and morphology of Li 2 O 2 towards enhanced Li-O 2 electrochemistry and the consequently improved electrochemical performance of the Li-O 2 battery. 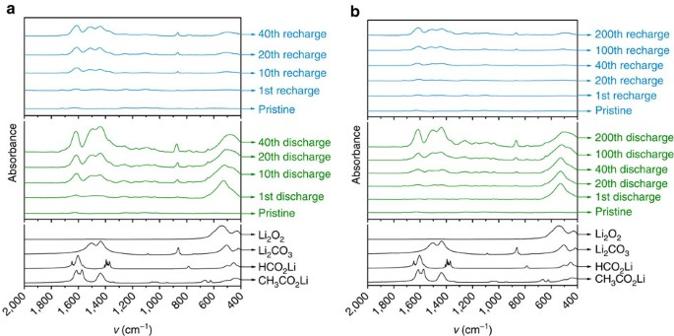Figure 7: Product composition. (a) SP cathode after different discharge–charge cycles. (b) P-HSC deposited onto CP cathode after different discharge–charge cycles. The spectra for Li2O2, Li2CO3, HCO2Li and CH3CO2Li are also shown for reference. Figure 7: Product composition. ( a ) SP cathode after different discharge–charge cycles. ( b ) P-HSC deposited onto CP cathode after different discharge–charge cycles. The spectra for Li 2 O 2 , Li 2 CO 3 , HCO 2 Li and CH 3 CO 2 Li are also shown for reference. Full size image In conclusion, we fabricated a P-HSC deposited onto CP cathode with a tailored hierarchically porous honeycomb-like structure by combining electrophoresis with a template replication method. We showed that a Li-O 2 cell composed of the P-HSC deposited onto CP cathode is capable of high-rate (5,900 mAh g − [1] at a current density of 1.5 A g −1 ) and long-term (100 cycles at a current density of 300 mA g −1 and a specific capacity limit of 1,000 mAh g −1 ) operation. The improvement is attributed to its tailored properties, which are vital to the operation of a Li-O 2 battery, including the unique porous structure with catalytically effective Pd NPs, high conductivity and the formation of isolated nanosheet-shaped discharge product Li 2 O 2 . Hence, we hope that the results presented here would encourage further studies of cathode design in Li-O 2 batteries, although many challenges in realizing practical devices still remain. Chemicals and materials Li 2 CO 3 , CH 3 CO 2 Li and HCO 2 Li were purchased from Sigma-Aldrich. Li 2 O 2 was purchased from Acros. Lithiated Nafion was purchased from the DuPont Company. CP was purchased from Torray. Ammonium hydroxide solution, ethanol, mercaptopropyltrimethoxysilane, tetraethylorthosilicate, palladium acetylacetonate, diethyl ether, sucrose, hydrofluoric acid, N -methyl-2-pyrrolidinone, TEGDME, LiCF 3 SO 3 and deuterium oxide were purchased from Aladdin Reagent. Toluene (C 7 H 8 ), acetone (C 3 H 6 O), and methanol (CH 3 OH) were purchased from Sinopharm Chemical Reagent Co. Ltd. P-HSC deposited onto CP cathode preparation The synthesis procedure for the SS was described by Stöber et al. [46] A 15-ml aliquot of a concentrated aqueous NH 4 OH solution was added into an aqueous ethanol solution (ethanol 200 ml, H 2 O 14 ml) and the resulting solution was stirred vigorously for 30 min. Then, 15 ml of tetraethylorthosilicate was added and the solution was stirred for 10 h. The mixture was centrifuged, decanted and dried at 100 °C. The surface of the SS was functionalized with MPS groups. Mercaptopropyltrimethoxysilane (6 ml) was added to 200 ml of a dried C 7 H 8 solution containing 2.0 g of SS, and the resulting mixture was refluxed at 110 °C for 12 h. The solution was cooled to room temperature and filtered, washed with C 7 H 8 , ether, C 3 H 6 O and CH 3 OH, and was dried at 50 °C. These MPS-SS were dispersed into a mixed solvent of C 3 H 6 O and CH 3 OH after ultrasonicating for 30 min. Electrophoretic deposition of the MPS-SS was performed in a beaker with a vertical CP anode and a stainless steel sheet as a counter cathode connected to a direct current power supply through an ammeter. The two electrodes were kept parallel at 1.0–1.5 cm apart in the suspension; a constant deposition voltage of 15–25 V was used for the electrophoretic deposition. The palladium precursor, palladium acetylacetonate, was then adsorbed onto the surface of the obtained MPS-SS deposited onto CP. This Pd 2+ -MPS-SS deposited onto CP was heated in an argon–hydrogen atmosphere at 250 °C for 1 h to produce Pd-MPS-SS deposited onto CP. Then, the obtained samples were soaked in a sucrose solution (20 wt%) for 20 min, and the excess solution was removed from the samples by filtration. The samples were dried at 70 °C for 3 h under vacuum and then calcined at 850 °C for 3 h under a nitrogen atmosphere. This composite was treated with 10 M hydrofluoric acid solution to remove SS. HSC deposited onto CP cathode preparation The HSC deposited onto CP cathode was prepared by a similar process to the P-HSC deposited onto CP cathode, except for the absence of Pd nanocrystals. Characterization The morphologies and structures of the materials were characterized using various physiochemical techniques, including PXRD, field emission scanning electron microscopy, TEM, nitrogen adsorption/desorption isotherms, thermogravimetric/differential thermal analysis and Raman spectra analysis. The discharge and recharge product were characterized using PXRD and FTIR spectroscopy. The electrolyte stability was determined by 1 H NMR analysis. Li-O 2 cell preparation and electrochemical measurements The electrochemical performance of the Li-O 2 cell was analysed using a 2025-type coin cell ( Supplementary Fig. S17 ). All of the cells were assembled in a glove box under an Ar atmosphere using a lithium metal foil anode, a glass fibre separator, an oxygen cathode and an electrolyte containing 1 M LiCF 3 SO 3 in TEGDME. The as-fabricated HSC deposited onto CP and P-HSC deposited onto CP electrodes was used as O 2 cathodes for the Li-O 2 cells. The conventional SP carbon cathode were prepared by coating homogenous ink composed of a mixture of 80 wt% SP carbon and 20 wt% lithiated Nafion onto the CP current collector. The galvanostatic discharge/charge tests were performed in a specific capacity-controlled mode at various current densities. The electrochemical impedance spectroscopy of the cell was evaluated using a BioLogic VMP3 electrochemical workstation within a frequency range of 10 6 to 10 −2 Hz. CV with a scan rate of 0.1 mV s −1 was also performed in the range of 2.6–4.3 V. Instrumentation PXRD measurements were performed on a Bruker D8 Focus power X-ray diffractometer with Cu K α radiation. SEM was performed on a field emission Hitachi S-4800 instrument operating at an accelerating voltage of 10 kV. Samples for SEM were prepared by dispersing the as-prepared product in ethanol by sonicating for ~5 min and then depositing onto an indium tin oxide glass attached to an SEM brass stub. TEM was performed using an FEI Tecnai G2 S-Twin instrument with a field emission gun operating at 200 kV. FTIR tests were performed on a Nicolet 6700 spectrometer. The Raman spectrum was collected using a micro-Raman spectrometer (Renishaw) with a 532-nm wavelength laser. Nitrogen adsorption measurements were performed on a Micromeritics ASAP 2020 adsorption analyser. Specific surface areas were calculated by the Brunaure–Emmert–Teller method. Pore volumes and sizes were estimated from the pore-size distribution curves from the adsorption isotherms using the Barrett–Joyner–Halenda method. 1 H NMR spectra were examined on a Bruker Avance II 400 spectrometer. The thermogravimetric/differential thermal analysis was performed at a heating rate of 2.5 °C in flowing air (NETZSCH5 STA 449F3, Germany). CV measurements were performed on a BioLogic VMP3 electrochemical workstation. Li-O 2 cell measurements were cycled on a LAND CT2001A multi-channel battery testing system. Electrochemical impedance spectroscopy was also performed on a BioLogic VMP3 electrochemical workstation over a frequency range from10 6 to 10 −2 Hz. How to cite this article: Xu, J.-J. et al. Tailoring deposition and morphology of discharge products towards high-rate and long-life lithium-oxygen batteries. Nat. Commun. 4:2438 doi: 10.1038/ncomms3438 (2013).